Microbiota-derived lactate accelerates colon epithelial cell turnover in starvation-refed mice Oral food intake influences the morphology and function of intestinal epithelial cells and maintains gastrointestinal cell turnover. However, how exactly these processes are regulated, particularly in the large intestine, remains unclear. Here we identify microbiota-derived lactate as a major factor inducing enterocyte hyperproliferation in starvation-refed mice. Using bromodeoxyuridine staining, we show that colonic epithelial cell turnover arrests during a 12- to 36-h period of starvation and increases 12–24 h after refeeding. Enhanced epithelial cell proliferation depends on the increase in live Lactobacillus murinus , lactate production and dietary fibre content. In the model of colon tumorigenesis, mice exposed to a carcinogen during refeeding develop more aberrant crypt foci than mice fed ad libitum . Furthermore, starvation after carcinogen exposure greatly reduced the incidence of aberrant crypt foci. Our results indicate that the content of food used for refeeding as well as the timing of carcinogen exposure influence the incidence of colon tumorigenesis in mice. The gastrointestinal (GI) tract must adapt to drastic changes in the lumenal environment to maintain homoeostasis, and responses to ingested food are the most fundamental physiological adaptations. Epithelial cells (EC) in the GI tract undergo rapid self-renewal, with a new gut lining produced approximately every 3 days [1] . However, the turnover rate is not always constant. For example, gut EC proliferation rates undergo circadian fluctuation in rodents [2] , [3] and humans [4] , [5] , which alters the morphology and function of the GI tract. In the normal human rectal biopsies, 3 H-thymidine incorporation into cells is higher at night and lower in the afternoon [5] . This circadian rhythm is controlled by clock genes in the central nervous system, as well as local expression of clock genes in intestinal tissue. EC proliferation rates also vary in a longer time span. For example, the GI tract of animals becomes atrophic during hibernation but undergoes rapid recovery on food intake after hibernation [6] , [7] . To illustrate, snakes usually eat after starvation of several months. On food intake, the snake intestine doubles in wet and dry mass within 1 day, largely as a result of a sixfold increase in microvillus length and a doubling of mucosal EC volume [8] . Thus, oral food intake should greatly change the rate of intestinal cell turnover. In nocturnal rodents, daytime feeding is a strong synchronizer of GI clock genes [9] . In rats, starvation reduces the weight and thickness of the small intestine [10] . In humans, total parenteral nutrition causes atrophy of intestinal mucosa [11] , [12] . Therefore, oral food intake is necessary for maintenance of cell proliferation and has the highest impact on the morphology and function of the GI tract. However, the mechanisms underlying how food intake regulates EC proliferation are not fully elucidated. In particular, there are few reports about how food intake affects colonic EC proliferation. Colonic EC turnover is slower than cell turnover in the small intestine. One reason may be the major difference in the luminal environments of the small and large intestines. Nutrients are mostly digested and absorbed in the small intestine, whereas the colon is colonized by microbiota. Thus, instead of orally ingested nutrients taken in by the host, the colon lumen is rich in microbial metabolites and fermentation products produced by the microbiota. As a result, colonic EC rely heavily on fermentation products of intestinal microorganisms, including butyric acid, as a source of carbon and energy [13] . The quality of nutrients for colonic EC is thus associated with the microbiota ‘enterotype’ [14] , [15] of the host and may also be associated with the incidence of diseases in the GI tract, including colorectal cancer, as well as diseases affecting other organs [16] . In this study, we found that starvation arrested colon EC turnover, and refeeding induced hyperproliferation in mice. The enhanced EC proliferation was dependent on the microbiota, more specifically lactobacilli and their metabolite lactic acid, which likely supported energy production in EC. We also found that this shift of EC turnover rate by starvation-refeeding dramatically changed the susceptibility to carcinogen exposure. Transient proliferation of colonic EC in refed mice We first evaluated the EC turnover of the small and large intestines on starvation and refeeding by quantifying bromodeoxyuridine (BrdU) incorporation into EC. After 36 h of starvation, the number of BrdU+ cells in both the small intestine and colon was less than in non-starved controls ( Supplementary Fig. S1a ), but the difference was only statistically significant in the colon ( Fig. 1a ). Cell turnover in the small intestine recovered to the level of non-starved control mice by 2 h after refeeding. In contrast, in the colon, recovery of cell proliferation was not seen until 6 h after refeeding; thereafter, proliferation exceeded control levels by approximately threefold at 12 h. This excessive cell proliferation continued for 24 h and returned to basal levels by 76 h after refeeding ( Fig. 1 ). In spite of the increased number of proliferating cells, there was no apparent change in the thickness of the colonic mucosa. However, the frequency of apoptosis detected with terminal deoxynucleotidyl transferase dUTP nick-end labelling (TUNEL) staining was not increased when compared with control mice fed ad libitum , whereas TUNEL + cells were very rare and found only in luminal surface EC ( Supplementary Fig. S1b ). This indicated that mucosal thickness did not change significantly because of an appropriately balanced rate of cell turnover, that is, enhanced proliferation with increased shedding rate of EC. This transient hyperproliferation of colonic EC was observed in several mouse strains, irrespective of gender or age ( Supplementary Fig. S2a–c ). We also found that starvation for only 12 h was sufficient to evoke the same refeeding-induced hyperproliferation response ( Supplementary Fig. S2d ). Thus, even transient starvation has a substantial impact on colonic EC turnover. Because a 12-h starvation period would be expected to occur on a daily basis, we also examined the daily changes in colonic EC proliferation without a controlled starvation period. As expected, considerable fluctuation in the number of BrdU+ cells was observed ( Supplementary Fig. S2e ). A high number of proliferating cells, comparable to the increased proliferation observed in refed mice, was seen at approximately noon in our facility. This observation does fit with mice being more active and feeding during the dark cycle and falling asleep (and presumably fasting) during the light cycle. 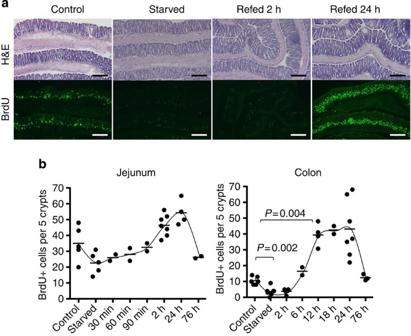Figure 1: Starvation-refeeding induced transient colonic EC hyperproliferation. (a) Colonic tissues were taken from mice fedad libitum(control), mice starved for 36 h and mice starved for 36 h and refed with normal bait (CE2) for 2 or 24 h. Frozen sections were stained with hematoxylin and eosin (H&E; upper) and anti-BrdU antibody (lower, green). Scale bar, 200 μm. (b) Number of BrdU+ cells per five crypts was counted at each time point. Each dot indicates an individual mouse. Mann–Whitney test was performed forP-value. Figure 1: Starvation-refeeding induced transient colonic EC hyperproliferation. ( a ) Colonic tissues were taken from mice fed ad libitum (control), mice starved for 36 h and mice starved for 36 h and refed with normal bait (CE2) for 2 or 24 h. Frozen sections were stained with hematoxylin and eosin (H&E; upper) and anti-BrdU antibody (lower, green). Scale bar, 200 μm. ( b ) Number of BrdU+ cells per five crypts was counted at each time point. Each dot indicates an individual mouse. Mann–Whitney test was performed for P -value. Full size image Because significantly increased EC proliferation was seen in the colon but not in the small intestine, we hypothesized that microbiota may be involved in the underlying mechanisms. Presence of microbiota stimulates innate immune responses through bacterial components, as well as fermentation products. To test the importance of the microbiota for EC proliferation responses to starvation-refeeding, mice were given oral antibiotics. Hyperproliferation in the colon was not observed in mice treated with antibiotics, although recovery of the small intestine was unaffected ( Fig. 2a ). As fermentation of dietary fibre depends on the action of microbiota, we also eliminated fibre from the mouse diet using a powdered formula of oral rehydration solution (ORS) containing glucose and salt, or an elemental diet containing dextran with amino acids and other nutritional supplements for refeeding after starvation. The small intestinal cell turnover in treated mice was similar to mice fed with normal bait (CE2). However, hyperproliferation in the colon did not take place in the absence of dietary fibre ( Fig. 2a ). The importance of microbiota in refeeding-induced colonic hyperproliferation was further confirmed in germ-free mice. In these mice, starvation-refeeding induced the transient decrease in BrdU + cells with subsequent recovery in the small intestine similar to that observed in specific pathogen-free (SPF) mice. However, the refeeding-induced colonic hyperproliferation was not observed in germ-free mice ( Fig. 2b ), consistent with the results obtained from SPF mice treated with antibiotics. From these results, we conclude that accelerated colonic EC turnover after starvation-refeeding is triggered by a microbiota-dependent mechanism. Lack of hyperproliferation in ORS or elemental diet refed mice suggests that degradation products of dietary fibre by live bacteria are required to support the hyperproliferation response. 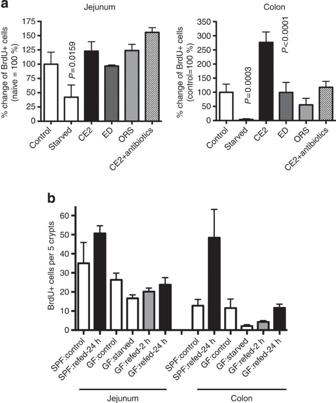Figure 2: Requirement for live microbiota and dietary fibre for refed-induced hyperproliferation. (a) Mice were starved for 36 h and refed with CE2, ED or ORS. A group of mice refed with CE2 was also given oral antibiotics. The percentage of BrdU+ cells per crypt in the colon 12 h after refeeding was compared (control=100%). Data are shown as an average+s.d. for 4–6 mice for each group. Statistically significant differences from the control group are indicated with aP-value (Mann–Whitney test). (b) Germ-free mice were starved for 36 h and refed CE2 for the indicated time. Data are shown as an average+s.d. for three mice for each group. Figure 2: Requirement for live microbiota and dietary fibre for refed-induced hyperproliferation. ( a ) Mice were starved for 36 h and refed with CE2, ED or ORS. A group of mice refed with CE2 was also given oral antibiotics. The percentage of BrdU+ cells per crypt in the colon 12 h after refeeding was compared (control=100%). Data are shown as an average+s.d. for 4–6 mice for each group. Statistically significant differences from the control group are indicated with a P -value (Mann–Whitney test). ( b ) Germ-free mice were starved for 36 h and refed CE2 for the indicated time. Data are shown as an average+s.d. for three mice for each group. Full size image Lactobacillus murinus induced accelerated EC turnover The importance of microbiota in refeeding-induced colonic hyperproliferation prompted us to investigate possible alterations in the composition of microbiota during starvation and refeeding. The number of bacteria decreased in both the small and large intestines after starvation. Bacterial numbers recovered to ~50% of baseline at 24 h in the small intestine of mice refed either CE2 or ORS. In contrast, the number of bacteria was approximately twofold greater in the colons of refed animals than in the colons of untreated controls ( Fig. 3a ). Thus, bacterial outgrowth occurred in the refed-phase concomitant with hyperproliferation in the colon. In fluorescence in situ hybridization (FISH) using a universal probe for the bacterial 16S rRNA sequence, overgrown bacteria adhered onto the surfaces of the EC, even in the deep pits of the crypts, which was not observed in control mice ( Fig. 3b ). However, bacterial translocation across the EC layer was not observed using FISH. The composition of the microbiota analyzed by denaturing gradient gel electrophoresis (DGGE) demonstrated that Lactobacillus murinus was a major species in the small intestines of control mice, which disappeared after starvation ( Supplementary Fig. S3 ). The bacterium related to Streptococcus alactolyticus was detected in the small intestines of animals starved or refed for 2 h, and L. murinus reappeared in either CE2- or ORS-refed mice. In the colon, appearance of L. murinus was detected only in CE2-refed mice but not in control, starved or ORS-refed mice ( Fig. 3c ). Further, starvation-refeeding experiments using gnotobiotic mice monoassociated with L. murinus showed that presence of L. murinus alone was able to reconstitute colonic EC hyperproliferation in refed mice ( Fig. 3d ). Thus, colonic EC hyperproliferation on refeeding seems tightly associated with the outgrowth of L. murinus. 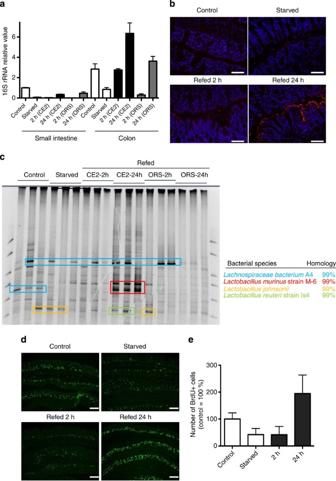Figure 3:  Colonic EC hyperproliferation is induced byLactobacillus murinus. (a) Number of bacteria determined by the 16S rRNA value. Mice were starved for 36 h and refed with the indicated formula in parentheses for the indicated time duration. Data are shown as an average+s.d. for three mice for each group. (b) FISH analysis of the starvation-refed colon with the 16S RNA probe. Scale bar, 100 μm. (c) DGGE analysis of colonic luminal contents in control mice and mice starved for 36 h and refed with CE2 or ORS for 2 or 24 h. Colonic luminal contents were collected and the microbial species determined, as described in the Methods. Each lane represents samples from individual mice. (d) Gnotobiotic mice were generated by inoculation ofLactobacillus murinusinto germ-free mice. Frozen sections were stained by anti-BrdU antibody (green). Scale bar, 200 μm. (e) Number of BrdU+ cells is shown as relative to control gnotobiotic mice. Data are shown as an average+s.d. for three mice for each group. Figure 3:  Colonic EC hyperproliferation is induced by Lactobacillus murinus. ( a ) Number of bacteria determined by the 16S rRNA value. Mice were starved for 36 h and refed with the indicated formula in parentheses for the indicated time duration. Data are shown as an average+s.d. for three mice for each group. ( b ) FISH analysis of the starvation-refed colon with the 16S RNA probe. Scale bar, 100 μm. ( c ) DGGE analysis of colonic luminal contents in control mice and mice starved for 36 h and refed with CE2 or ORS for 2 or 24 h. Colonic luminal contents were collected and the microbial species determined, as described in the Methods. Each lane represents samples from individual mice. ( d ) Gnotobiotic mice were generated by inoculation of Lactobacillus murinus into germ-free mice. Frozen sections were stained by anti-BrdU antibody (green). Scale bar, 200 μm. ( e ) Number of BrdU+ cells is shown as relative to control gnotobiotic mice. Data are shown as an average+s.d. for three mice for each group. Full size image Lactate and L. murinus -induced EC hyperproliferation To identify the inducer of colonic EC hyperproliferation, we attempted to reconstitute hyperproliferation in ORS-refed mice. As shown in Fig. 4a , we first confirmed that intrarectal injection of fresh caecal contents from starvation-CE2-refed mice into ORS-refed mice fully induced hyperproliferation, demonstrating that intestinal luminal contents are critical for the hyperproliferation response. Rectal administration of ultraviolet-killed total flora or L. murinus (1 × 10 10 colony-forming units, 0.1 ml per mouse) only partially reconstituted CE2-refed hyperproliferation, suggesting that live bacterial metabolites may be required for the full response. To identify the hyperproliferation-inducing factor(s), metabolome analysis of the colonic luminal contents was performed using a gas chromatography–mass spectrometry (GC–MS) system ( Supplementary Fig. S4 ). Some amino acids were markedly decreased in starved mice and recovered to control levels on refeeding with either CE2 or ORS, except aspartic acid, asparagines and glutamine, which did not return to control levels in ORS-refed mice. We found that organic acids were classified into at least two groups according to the pattern of alteration during starvation-refeeding. One group increased in CE2-refed mice but not in ORS-refed mice, which included lactic acids, glycolic acid, 3-hydroxypropanoic acid, maleic acid, glutaric acid, 2-deoxytetronic acid, 3-hydroxyphenylacetic acid and 4-hydroxybenzoic acid. The second group increased in starved mice and decreased after CE2-refeeding but not after ORS-refeeding, and included caproic acid, 2-hydroxybutyric acid, 2-hydroxyisovaleric acid, 4-hydroxyphenylacetic acid and malonic acid. Representative organic acids of these two groups are shown in Fig. 4b . Most fatty acids analyzed and urea showed similar kinetic patterns to the second group of organic acids ( Supplementary Fig. S4 ). As we found that live Lactobacillus and its metabolite(s) were required for colonic EC hyperproliferation, we hypothesized that organic acids that increased on refeeding (that is, the first group) were most likely associated with EC hyperproliferation. On the basis of the total ion peak values of the GC–MS analysis ( Supplementary Fig. S5a ) and a separate analysis of luminal contents using NMR from control mice ( Supplementary Fig. S5b ), the composition of organic acid was estimated. According to these results, a mixture containing acetic acid, propionic acid, butyric acid, lactic acid, 3-hydroxypropionic acid, glycolic acid, succinic acid and glyceric acid was tested for its ability to support EC hyperproliferation on refeeding. This mixture induced hyperproliferation (that is, increased the number of BrdU + cells) more efficiently than ultraviolet-killed L. murinus , and co-administration of this mixture with killed bacteria induced the full hyperproliferative response ( Fig. 4a ). As L. murinus produces mainly lactate, we treated ORS-refed animals with 500 mM lactate alone rectally and examined colonic EC proliferation. Lactate alone resulted in EC hyperproliferation comparable to that of the organic acid mixture, indicating that this component was largely responsible for the observed response. To further confirm the action of lactic acid, mice refed with CE2 were treated orally and rectally with antibiotics and either lactate, butyrate, acetate, 3-hydroxypropanoate and succinate. As shown in Fig. 4a , only lactate induced EC hyperproliferation on refeeding, and deletion of lactate from the organic acid mixture resulted in the loss of hyperproliferation. This indicated that lactate was the most important organic acid for stimulation of colonic EC turnover in response to starvation-refeeding. Indeed, in germ-free mice, there were no significant changes in the amount of lactic acid during starvation-refeeding, while increased lactic acid was evident in the cecums and colons of L. murinus -monoassociated mice on refeeding ( Fig. 4c ). Glycolic acid, which also increased in the refed colons of SPF mice ( Fig. 4b ), did not change significantly on starvation-refeeding in germ-free mice and there were no differences in the levels of glycolic acid between germ-free and L. murinus -monoassociated mice. In summary, outgrowth of L. murinus and, therefore, production of lactic acid, induced the hyperproliferation of colonic EC. To further confirm this finding, we prepared gnotobiotic mice monoassociated with lactate-producing Bifidobacterim longum subsp. infantis ( B. infantis ) and non-lactate-producing Bacteroides thetaiotaomicron ( B. thetaiotaomicron ) [17] , [18] . As shown in Fig. 4d , starvation-refed B. infantis -monoassociated mice demonstrated hyperproliferation at refeeding. On the other hand, B. thetaiotaomicron did not induce hyperproliferation. These results clearly demonstrate that a bacterial metabolite (lactate) rather than bacterial components has a major role to induce accelerated cell turnover. 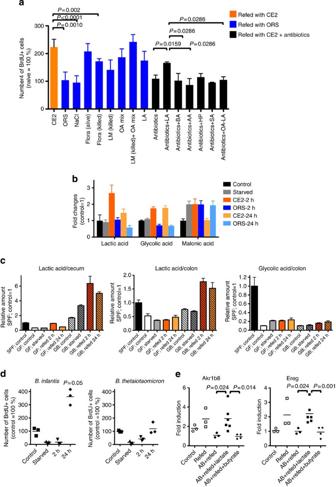Figure 4: Lactate is required for hyperproliferation. (a) Mice were starved for 36 h and refed CE2 (orange) or ORS (blue) or CE2 with oral antibiotics (black) for 12 h. In ORS-refed mice, the number of BrdU+ cells in the colon without rectal injection (ORS), with rectal injection of control 500 mM NaCl (NaCl), fresh caecal contents from CE2-refed mice (flora-alive), killed flora (flora-killed), killedL. murinus(LM-killed), organic acid mixture (OA mix), LM-killed plus organic acid mixture (LM-killed+OA mix), 500 mM lactate (LA) or a combination of these are shown. In mice refed with CE2 and treated with oral antibiotics, 500 mM NaCl (antibiotics), lactate (LA), butyrate (BA), acetate (AA), 3-hydroxypropionate (HP), succinate (SA) or OA mixture minus lactate (OA−LA) was administered intrarectally together with antibiotics three times during refeeding. Data are shown as the average+s.d. of 3–7 mice relative to control (fedad libitum) mice. (b) Typical patterns of metabolome analysis as relative changes from the control condition. Data are shown as the average +s.d. of three mice as the relative signal intensity to control SPF mice. (c) Relative amount of lactic acid in the caecum and colon, and glycolic acid in the colon from starvation-refed, germ-free (GF) and gnotobiotic mice monoassociated withL. murinus(GB, hatched). Data are shown as the mean+s.d. of three mice as the relative signal intensity to control SPF mice. (d) Number of BrdU+ cells in the colon of gnotobiotic mice monoassociated with lactate-producingBifidobacterim infantisor non-lactate-producingBacteroides thetaiotaomicronshown as % of control (fedad libitum). Short bar indicates the mean value. (e) Gene expression in the colon. Mice were starved for 36 h and refed CE2. Some mice were treated with oral antibiotics (AB), and 500 mM lactate or butyrate was administered intrarectally together with antibiotics three times during refeeding. After 12 h of refeeding, distal 1/3 of the colon was subjected to total RNA extraction and quantitative RT–PCR for Akr1b8 and Ereg. Data were shown as relative expression (AB+refed=1). Each dot represents individual mice, and short bar indicates the mean value. In panelsa,dande,P-values were calculated using Mann–Whitney test. Figure 4: Lactate is required for hyperproliferation. ( a ) Mice were starved for 36 h and refed CE2 (orange) or ORS (blue) or CE2 with oral antibiotics (black) for 12 h. In ORS-refed mice, the number of BrdU+ cells in the colon without rectal injection (ORS), with rectal injection of control 500 mM NaCl (NaCl), fresh caecal contents from CE2-refed mice (flora-alive), killed flora (flora-killed), killed L. murinus (LM-killed), organic acid mixture (OA mix), LM-killed plus organic acid mixture (LM-killed+OA mix), 500 mM lactate (LA) or a combination of these are shown. In mice refed with CE2 and treated with oral antibiotics, 500 mM NaCl (antibiotics), lactate (LA), butyrate (BA), acetate (AA), 3-hydroxypropionate (HP), succinate (SA) or OA mixture minus lactate (OA−LA) was administered intrarectally together with antibiotics three times during refeeding. Data are shown as the average+s.d. of 3–7 mice relative to control (fed ad libitum ) mice. ( b ) Typical patterns of metabolome analysis as relative changes from the control condition. Data are shown as the average +s.d. of three mice as the relative signal intensity to control SPF mice. ( c ) Relative amount of lactic acid in the caecum and colon, and glycolic acid in the colon from starvation-refed, germ-free (GF) and gnotobiotic mice monoassociated with L. murinus (GB, hatched). Data are shown as the mean+s.d. of three mice as the relative signal intensity to control SPF mice. ( d ) Number of BrdU+ cells in the colon of gnotobiotic mice monoassociated with lactate-producing Bifidobacterim infantis or non-lactate-producing Bacteroides thetaiotaomicron shown as % of control (fed ad libitum ). Short bar indicates the mean value. ( e ) Gene expression in the colon. Mice were starved for 36 h and refed CE2. Some mice were treated with oral antibiotics (AB), and 500 mM lactate or butyrate was administered intrarectally together with antibiotics three times during refeeding. After 12 h of refeeding, distal 1/3 of the colon was subjected to total RNA extraction and quantitative RT–PCR for Akr1b8 and Ereg. Data were shown as relative expression (AB+refed=1). Each dot represents individual mice, and short bar indicates the mean value. In panels a , d and e , P -values were calculated using Mann–Whitney test. Full size image Upregulation of energy production pathway in refed colon EC To characterize the signature of hyperproliferative EC induced by refeeding, we compared the gene expression profiles of purified EC derived from refed mice and refed mice treated with antibiotics. Pathway analysis showed that genes increased 1.5-fold in refed EC than in refed EC treated with antibiotics indicated the enrichment of the genes related to energy production, lipid metabolism, small-molecule biochemistry as the top networks, and glycerolipid metabolism as the top canonical pathway as shown in Tables 1 and 2 and in Supplementary Figs S6 and S7 . This finding indicates that refed EC actively produce energy using stored fat. The glycerolipid metabolism pathway shown in Supplementary Fig. S7 clearly indicated increased fatty acid release from glycerolipids. The fatty acids that underwent beta-oxidation into acetyl CoA can eventually enter the tricarboxylic acid cycle to produce ATP, suggesting that the presence of luminal lactate facilitates ATP production through enhanced use of lipids. Table 1 Top five gene networks of 1.5-fold upregulated genes in colonic EC from refed mice compared with refed mice treated with antibiotics. Full size table Table 2 Top five canonical pathways of 1.5-fold upregulated genes in colonic EC from refed mice compared with refed mice treated with antibiotics. Full size table To confirm that this gene expression profile is related to lactate in the lumen, we attempted to validate the result with quantitative PCR with reverse transcription (RT–PCR) using fresh colon exposed to lactate. Akr1b8, encoding aldo-keto reductase family 1, member B8, listed as enzyme commission number 1.1.1.21 in Supplementary Fig. S7 , was one of top 10 genes enriched in refed colon ( Supplementary Fig. S8 ). Ereg encodes epiregulin, a member of epidermal growth factor family and 1.7-fold higher in refed colon than that treated with antibiotics ( Supplementary Fig. S8 ). As shown in Fig. 4e , both gene levels tended to be higher in refed mice than those of mice fed ad libitum (control). This upregulation was not seen in refed mice treated with antibiotics; However, additional rectal injection of lactate significantly upregulated both genes. Butyrate failed to induce expression of these genes in antibiotic-treated mice. These results further support the notion that lactate changes the gene expression of EC and drives metabolic shift to enhance cell proliferation in refed mice. Starvation-refeeding alters susceptibility to carcinogen Our observation that colonic EC turnover is accelerated after starvation-refeeding in the presence of microbiota prompted us to test whether this proliferative response to refeeding sensitizes colonic EC to tumorigenesis. To this end, we employed a mouse model of tumorigenesis using the chemical carcinogen azoxymethane (AOM), which induces aberrant crypt foci (ACF) of the colon. The experimental protocol is illustrated in Supplementary Fig. S9 . In mice given AOM 8 h after the initiation of refeeding, at the beginning of hyperproliferation of the colon, the number of ACF was significantly higher than in mice fed ad libitum ( Fig. 5a ). In contrast, when mice were challenged with AOM followed by starvation and refeeding, it resulted in a striking decrease in the number of ACF ( Fig. 5a ). In addition to ACF, the colonic mucosa of refed-plus AOM mice appeared rough and scraggly ( Fig. 5b ), matching the histological image, in which the deformed and atypical shapes of the crypts were scattered ( Fig. 5c ); however, crypts of mice with AOM followed by starvation had a smooth appearance ( Fig. 5b ) lined with goblet cells ( Fig. 5c ). As we thought that hyperproliferation was responsible for the increased number of ACF in refed-plus AOM mice, oral antibiotics were administered to AOM-treated mice during refeeding to block the production of lactic acid by L. murinus and thereby prevent EC hyperproliferation. This treatment reduced the number of ACF to that of control mice and decreased the irregularities observed in the colonic mucosa ( Fig. 5a ). These observations suggest that hyperproliferation in response to refeeding increases the number of AOM-susceptible cells, resulting in a greater number of ACF. In contrast, accelerated cell turnover after temporal starvation appears to eliminate damaged cells efficiently. Although AOM metabolism may drastically change during starvation and refeeding, expression levels of CYP2E1, a major enzyme associated with the activation of AOM, did not correlate with the number of ACF ( Supplementary Fig. S9b ). We think the metabolic rate of AOM is not a major factor that distinguishes sensitivity to DNA damage between starved and refed mice ( Supplementary Discussion ). 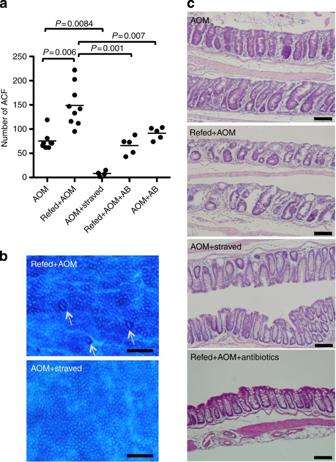Figure 5: Effects of starvation-refeeding on exposure to carcinogen. (a) The number of ACF in the colon. AOM, mice fedad libitumand treated with AOM; Refed+AOM, treatment with AOM at refeeding; AOM+starved, mice fedad libitumand treated with AOM, then starvation was begun on the following day; Refed+AOM+AB, refed+AOM mice were treated with oral antibiotics; AOM+AB, mice were fedad libitumand treated with AOM and oral antibiotics. These treatments were repeated five times a week. A week after the last injection of AOM, ACF in the colon were quantified. Each dot indicates an individual mouse.P-values were calculated using Mann–Whitney test. For a detailed protocol, seeSupplementary Fig. S9. (b) Methylene blue staining of the colon from Refed+AOM or AOM+starved mouse groups. Arrows indicate ACF. Images were captured with a stereomicroscope. Scale bar, 0.5 mm. (c) Formalin-fixed paraffin-embedded sections were stained with H&E. Scale bar, 100 μm. All images were taken from the same region of the colon (distal one-third). Figure 5: Effects of starvation-refeeding on exposure to carcinogen. ( a ) The number of ACF in the colon. AOM, mice fed ad libitum and treated with AOM; Refed+AOM, treatment with AOM at refeeding; AOM+starved, mice fed ad libitum and treated with AOM, then starvation was begun on the following day; Refed+AOM+AB, refed+AOM mice were treated with oral antibiotics; AOM+AB, mice were fed ad libitum and treated with AOM and oral antibiotics. These treatments were repeated five times a week. A week after the last injection of AOM, ACF in the colon were quantified. Each dot indicates an individual mouse. P -values were calculated using Mann–Whitney test. For a detailed protocol, see Supplementary Fig. S9 . ( b ) Methylene blue staining of the colon from Refed+AOM or AOM+starved mouse groups. Arrows indicate ACF. Images were captured with a stereomicroscope. Scale bar, 0.5 mm. ( c ) Formalin-fixed paraffin-embedded sections were stained with H&E. Scale bar, 100 μm. All images were taken from the same region of the colon (distal one-third). Full size image In this study, we found that transient starvation enhanced EC turnover on refeeding, and this response was dependent on the presence of commensal lactobacilli and its metabolite, lactate. We also found that carcinogen sensitivity was significantly increased during refeeding and was reduced by starvation after exposure to the carcinogen. There are a limited number of studies on colonic EC turnover during starvation. Using the metaphase-arrest technique, it has been reported that there is reduced ‘crypt cell production’ during starvation and an ‘overshooting’ recovery after refeeding [2] ; in rats, colonic EC responses are dependent on the presence of fermentable fibre [19] . Taken together with our results, these data indicate that our observations are not particular to our animal facility or animals colonized with certain microbiota. In this study, we identified lactic acid-producing L. murinus as the causal factor for the refeeding EC hyperproliferation response. As discussed below, because lactate was sufficient to accelerate EC turnover, many lactic acid-producing bacteria have the potential to induce a similar effect. In our study, L. murinus was detected in control (fed ad libitum ) conditions in the small intestine but was not a dominant strain in the colon at steady state. In some individual control mice, L. murinus was a major strain in the small intestine. In contrast, outgrowth of L. murinus was universally observed in the colons of refed mice. When the results of Fig. 3a–c are considered, L. murinus appeared to be the major constituent of refed colonic microbiota, apparently heavily attached to the mucosal surface. While L. murinus did reside in the small intestine before starvation, its outgrowth in the colon on starvation-refeeding was likely due to the luminal environment becoming particularly suitable for its growth. Colonization of L. murinus may be affected by changes in available nutrients, oxygen concentration, or host and microbial factors for adhesion, such as production and carbohydrate structure of host mucins, secretion of host antibacterial peptides and upregulation of microbial adhesins, including mucus-binding protein [20] . Indeed, luminal nutrients changed dramatically during starvation, and loss of villi in the small intestine reduced the available surface area for bacterial adhesion. All these changes may have favored the growth of L. murinus in the refed colon. Refeeding with ORS provides glucose as the energy source, which may not reach the colon lumen, sustains morphological recovery of small intestine EC. However, ORS-refeeding failed to support L. murinus colonization or hyperproliferation of colonic EC. In the experiment using gnotobiotic mice, we showed that monoassociation with L. murinus was sufficient to induce colonic EC hyperproliferation in refed mice. Therefore, we conclude that outgrowth of L. murinus induced colonic EC hyperproliferation on refeeding. In subsequent experiments, we identified lactate as the most important L. murinus metabolite for the induction of colon hyperproliferation. This conclusion is based on several pieces of evidence. First, metabolome analyses indicated that lactic acid levels increased substantially in the colons of CE2-refed animals but not in ORS-refed colons. Second, gnotobiotic mice monoassociated with L. murinus had contained elevated lactic acid levels in the colon, and gnotobiotic mice monoassociated with a lactate-producing stain but not a non-lactate-producing strain showed hyperproliferation after starvation. Third, in animals treated with antibiotics to eliminate normal flora, rectal administration of lactic acid but not butyrate or acetate supported colonic EC proliferation. This result surprised us, because butyrate and acetate are also major fermentation products of microbiota, and there is a wide range of evidence supporting their beneficial protective effects on colonic EC [21] , [22] , [23] , [24] , [25] . On the other hand, lactate has long been considered a dead-end waste product; however, some recent studies have shown that lactate has diverse metabolic and regulatory properties, such as being an energy source, a modulator of energy production, and a signalling molecule for cell repair and angiogenesis (reviewed in [26] ). Further, survival and function of some types of cells such as neurons and germ cells that demand high energy depend on the extracellular lactate provided by adjacent nursing cells, astrocytes and Sertoli cells [27] . Although we did not obtain direct evidence that lactate itself is used as an energy source, we speculate that the modified redox status of EC by starvation-refeeding might enable EC to respond to luminal lactate to promote energy production. On the basis of these observations, we posed the question, ‘What is the significance of colonic hyperproliferation on refeeding to health and disease?’ Treatment of refed animals with AOM clearly demonstrated that exposure to a carcinogen during the colonic hyperproliferation response to refeeding significantly increased the risk of tumorigenesis. In contrast, colonic hyperproliferation induced after exposure to a carcinogen appears to eliminate damaged cells efficiently. In general, starvation or calorie restriction has been reported to extend the lifespan of most species, including rodents and primates. The molecular basis for this observation has been proposed to be sirtuins and the nutritional signalling target of rapamycin pathway [28] , [29] . Studies also have shown that calorie restriction decreases the risk of colon cancer [30] ; however, our study suggests that the timing of carcinogen exposure is a critical factor. After transient starvation, there is a window of time when colonic EC become susceptible to DNA damage, and this greatly depends on the bacterial flora and luminal metabolite composition. Thus, our results provide new insight into the relationship between carcinogenesis, food intake and lifestyle. Mice Six-week-old male BALB/c mice were used for all experiments, unless otherwise indicated. All mice were obtained from CLEA Japan Inc. (Tokyo, Japan), maintained under SPF conditions at the National Center for Global Health and Medicine facility (Tokyo, Japan), and fed normal bait (CE2, Clea Japan). Germ-free mice (BALB/c background) were purchased from Sankyo Labo Service Corporation, Inc. and kept in an animal facility in RIKEN. All experiments were performed according to the Institutional Guidelines for the Care and Use of Laboratory Animals in Research and the approval of the local ethics committee at the National Center for Global Health and Medicine and RIKEN. Starvation and refeeding During starvation, mice were kept in plastic cages with bedding chips and drinking water without bait. Irrespective of the length of the starvation period, the refeeding period was set to begin at 8:00 in all experiments. Elementary diet (Elental) was obtained from Ajinomoto Co. Inc.. Powdered formula of ORS contained 675 g glucose, 130 g NaCl, 145 g trisodium citrate dihydrate and 75 g KCl mixed in a sterilized mortar. To eliminate endogenous flora, a 0.2-ml solution of 500 mg l −1 metronidazol and 1 g l −1 vancomycin was administered daily by oral–gastric gavage. After starvation, 12- and 24-h refeeding with elemental diet or ORS were able to recover body weights comparable to CE2. In enema experiments, ultraviolet irradiation-killed L. murinus was prepared, and pelleted cells were re-suspended in PBS (1 × 10 10 colony-forming units; 0.1 ml per mouse). For intrarectal administration of the reagents, 0.1 ml of the indicated solution was injected into the rectum three times within the first 12 h of refeeding (0, 4 and 8 h after refeeding), and animals were lightly anesthetized using inhaled sevoflurane. The organic acid mixture contained 600 mM acetic acid, 200 mM propionic acid, 200 mM butyric acid, 200 mM lactic acid, 200 mM 3-hydroxypropionic acid, 100 mM glycolic acid, 40 mM succinic acid and 200 mM glyceric acid (final concentrations). In some experiments, antibiotics (50 mg l −1 metronidazol and 0.1 g l −1 vancomycin, final concentration) were added to the solutions for rectal injection. Microbiological analysis 16S rRNA Bacterial genomic DNA was isolated as described previously with some modifications [31] . In brief, faecal samples were freeze-dried, homogenized, disrupted using 0.1-mm Zirconia/Silica Beads, and extracted with 10% sodium dodecyl sulphate/Tris-HCl plus ethylenediamine tetraacetic acid (EDTA) buffer solutions. Bacterial genomic DNA was purified from the faecal extracts using a phenol/chloroform/isoamyl alcohol method. Bacterial genomic DNA samples were amplified using SYBR premix Ex Taq (TAKARA BIO, Otsu, Japan) and universal primers for the genes encoding bacterial 16S rRNA [22] , [32] . The results were calculated as the amount relative to copy number detected in the small intestinal contents of control mice. DGGE analysis Bacterial genomic DNA samples were amplified by PCR with universal bacterial primers 954f and 1396r specific for the V6 to V8 regions of the 16S rRNA gene [33] . The reaction mixtures and PCR conditions were described previously [32] . After confirmation of the PCR product by agarose gel electrophoresis, DGGE was performed with the DCode universal mutation detection system (Bio-Rad Lab., Irvine, CA). Polyacrylamide gel conditions for the denaturing gradient, migration, and differentiation were described previously [33] . Electrophoresis was conducted with a constant voltage of 82 V at 60 °C for 15 h. Gels were stained with SYBR Green I (Lonza, Rockland, ME) and acquired by GelDoc XR (Bio-Rad Lab) [31] . Fluorescence in situ hybridization Bacterial 16s rRNA FISH was performed as described previously [34] . In brief, colonic tissue sections were fixed in 4% paraformaldehyde, washed in PBS, incubated in 50 μl of 30% formamide hybridization buffer containing 25 ng of 5′-Cy3-labelled universal oligonucleotide probes for eubacteria (EUB338, 5′-GCTGCCTCCCGTAGGAGT-3′) or the non-bacterial control (NONEUB, 5′-ACTCCTACGGGAGGCAGC-3′) for 90 min at 46 °C, and washed with the same stringency for 20 min at 48 °C. Stained sections were imaged on a DM-IRE2 confocal laser-scanning microscope (Leica Microsystem). Metabolome-GC/MS analysis and data processing Intestinal contents were collected and lyophilized. To extract low-molecular-weight metabolites, 10 mg of lyophilized intestinal contents were transferred to a clean tube and homogenized in 1,000 μl solvent mixture (MeOH:H 2 O:CHCl 3 =2.5:1:1). Then, 10 μl of 0.5 mg ml −1 2-isopropylmalic acid (Sigma-Aldrich, Tokyo, Japan) dissolved in distilled water was added to each tube, and the mixture was mixed well. The mixture was shaken at 1,200 r.p.m. for 30 min at 37 °C before being centrifuged at 16,000 g for 3 min at 4 °C. Nine-hundred microliters of the resultant supernatant were collected into a clean tube. Four-hundred fifty microliters of CHCl 3 were added to the collected supernatant and centrifuged at 16,000 g for 3 min at 4 °C, and 500 μl of supernatant were collected in a clean tube. Two-hundred microliters of distilled water were added to the collected supernatant and centrifuged at 16,000 g for 3 min at 4 °C; 500 μl of supernatant were collected in a clean tube. The collected supernatant was lyophilized using a freeze-dryer before oximation and the following derivatization. For oximation, 80 μl of 20 mg ml −1 methoxyamine hydrochloride (Sigma-Aldrich), dissolved in pyridine, was mixed with a lyophilized sample before being shaken at 1,200 r.p.m. for 90 min at 30 °C. Next, 40 μl N -methyl- N -trimethylsilyl-trifluoroacetamide (GL Science, Tokyo, Japan) were added for derivatization, and the mixture was incubated at 1,200 r.p.m. for 30 min at 37 °C. The mixture was centrifuged at 16,000 g for 5 min at 4 °C, and the resultant supernatant was subjected to GC–MS analysis. According to our previous reports [35] , [36] , GC–MS analysis was performed using GCMS-QP2010 Plus (Shimadzu Co., Kyoto, Japan) with a DB-5 column (30 m × 0.25 mm inner diameter; film thickness is 1.00 μm, J&W Scientific, Folsom, CA) and GCMS-QP2010 Ultra (Shimadzu Co., Kyoto, Japan) with a CP-SIL 8 CB low-bleed/MS column (30 m × 0.25 mm inner diameter, film thickness is 0.25 μm, Agilent Co., Palo Alto, CA). Processing of data obtained from GCMS-QP2010 Plus and GCMS-QP2010 Ultra was carried out as described previously [35] , [36] . For semi-quantification, the peak heights of each ion were calculated and normalized using the peak height of 2-isopropylmalic acid as an internal standard. Metabolome-NMR analysis NMR-based metabolomics was performed as described previously with minor modifications [37] . In brief, faecal metabolites from mice were extracted by gentle shaking with 100 mM potassium phosphate buffer containing 90% deuterium oxide and 1 mM sodium 2,2-dimethyl-2- silapentane-5-sulfonate as the chemical shift references ( δ =0.0 p.p.m. ), and analyzed by 1 H-NMR and 1 H, 13 C-NMR. Metabolite annotations were performed using our standard database [38] . Induction of ACF As shown in Supplementary Fig. S9 , mice were divided into five groups. Group 1 (AOM) was fed ad libitum and intraperitoneally injected with AOM (Sigma-Aldrich, 10 mg kg −1 ). Group 2 (refed+AOM) was starved for 24 h, refed with CE2 and injected with AOM 8 h after refeeding. Group 3 (AOM+starved) was injected with AOM at 16:00; fasting for 24 h was begun at 8:00 on the following day. Group 4 (refed+AOM+AB) was treated similar to Group 2 but oral antibiotics were administered, as described above, beginning with a 5-day starvation period. Group 5 (AOM+AB) was fed ad libitum , injected with AOM and given oral antibiotics for 5 days. These protocols were repeated weekly, five times. All mice groups were given AOM injections at 16:00. On day 37, colon tissues were obtained, washed and extended by flushing with PBS. Colons were opened longitudinally, fixed with formalin and stained with 3% methylene blue. ACF were enumerated under a stereomicroscope [39] . Gene expression profiling of colon ECs For global gene expression profiling in EC, colon tissues were stirred in 6.5 mM dithiothreitol in Hank's Balanced Salt Solution for 15 min at room temperature and in 10 mM EDTA in Hank's Balanced Salt Solution for 10 min. Treatment with EDTA was repeated 4–6 times until EC were released from the stroma. Single-cell suspensions of EC were stained with 7-amino-actinomycin D, fluorescein isothiocyanate-anti-CD45 and phycoerythrin-anti-EpCAM antibodies (BD). Viable EpCAM + CD45 − cells were sorted as purified EC (Moflo, Beckman Coulter, Tokyo, Japan). Total RNA was extracted according to standard protocols (Affymetrix). Targets were prepared and hybridized to the GeneChip Mouse Gene 1.0 ST Array (Affymetrix) according to standard protocols. GeneChip data sets were analyzed using GeneSpring GX 11 (Agilent). Array data were normalized using robust multi-array analysis algorithms. Statistical analysis All data are presented as the mean±s.d., unless indicated in the legend. For comparison of two groups, a non-parametric method (Mann–Whitney test) and Student’s t -test were used in comparisons as indicated in the legends. Results were determined as significant when P -values were less than 0.05. Statistical analyses were performed using GraphPad Prism 4 software (GraphPad Software, Inc). Methods for histological analyses, quantitative RT–PCR, and pathway analysis of gene expression profiling are described in the Supplementary Information . Accession codes: microarray data have been deposited in the Gene Expression Omnibus database under accession code GSE40370 . How to cite this article : Okada, T. et al . Microbiota-derived lactate accelerates colon epithelial cell turnover in starvation-refed mice. Nat. Commun. 4:1654 doi: 10.1038/ncomms2668 (2013).